Complete information acquisition in dynamic force microscopy Scanning probe microscopy has emerged as a primary tool for exploring and controlling the nanoworld. A critical part of scanning probe measurements is the information transfer from the tip–surface junction to the measurement system. This process reduces responses at multiple degrees of freedom of the probe to relatively few parameters recorded as images. Similarly, details of dynamic cantilever response at sub-microsecond time scales, higher-order eigenmodes and harmonics are lost by transitioning to the millisecond time scale of pixel acquisition. Hence, information accessible to the operator is severely limited, and its selection is biased by data processing methods. Here we report a fundamentally new approach for dynamic Atomic Force Microscopy imaging based on information–theory analysis of the data stream from the detector. This approach allows full exploration of complex tip–surface interactions, spatial mapping of multidimensional variability of material’s properties and their mutual interactions, and imaging at the information channel capacity limit. The rapid emergence of Scanning Probe Microscopy (SPM) techniques in the last three decades opened a new chapter in nanoscale exploration and manipulation by thousands of research groups worldwide [1] , [2] . The basic premise of SPM—a combination of localized, often atomic sized, probe and a detection system linking it to the macroscopic world allowed information on electronic [3] , mechanical [4] , magnetic [5] , electrostatic [6] , [7] and electromechanical [8] , [9] , [10] properties to be visualized at nanometre scales and in some cases with atomic resolution. In a broader sense, SPM imaging can be represented as an information channel [11] between the dynamic processes at the tip–surface junction and an observer via a data acquisition and processing system that convey the information on local properties and structure as probed through the tip–surface interactions. Correspondingly, progress in SPM techniques requires a synergy of improvements on multiple fronts, including microscope platforms, probes and the data acquisition process. In the last three decades, much attention has been focused on the development of low noise microscope platforms and high-quality probes, minimizing noise in the data acquisition process. Similarly, magnetic or chemical probe functionalization has been developed to allow for increased selectivity towards chosen interactions. However, relatively little effort has been devoted to improvements in information transfer. Indeed, the fundamental component of all force-based dynamic Atomic Force Microscopy (AFM) methods is the nexus between data processing electronics operating at millisecond time scales of pixel acquisition, and the sub-microsecond scale of cantilever oscillations. In such a process, multidimensional dynamic information of a vibrating cantilever is severely compressed to only several measured parameters. While for linear systems such representation is justified, real-world complications include distributed response of cantilever, as well as mode couplings, non-linearities and response transients. All of these contain detailed information on local sample properties that cannot be ignored or effectively compressed. The amount and quality of information obtained hence depends not only on the resolution of the microscope, but also internal distortions and channel noise during the information flow. Furthermore, the choice of information conversion scheme imposes the external observer bias on recorded data, for example, heterodyne detection in classical lock-in (LI) and phase-locked loop processing inevitably restricts physics of tip–surface interactions to purely sinusoidal processes. Notably, this limitation is recognized by the AFM community, and numerous techniques based on the detection of higher harmonics [12] , [13] and full force–distance curve measurements are being introduced to fully capture behaviour of a tip–surface interactions. The advantage of multiple modulation techniques have further extended the spectrum of these methods [14] . However, in all cases the detected signal contains multiple harmonics of response, at different time scales, from which materials-specific interactions can be reconstructed only with complex inversion procedures [15] , [16] . Furthermore, the serendipitous information in transient responses and single events, generally remains unrecognized and ignored. Here we introduce a novel principle for information acquisition and processing in dynamic AFM techniques, further referred to as general mode (G-mode) SPM, based on information–theory analysis of the cantilever output stream. This approach is based on full acquisition of the cantilever position data during an experiment and subsequent multivariate statistical analyses of the full trajectory data set, yielding statistically relevant components of response and their spatial variability. This approach allows one to examine and store only statistically relevant components of cantilever response and hence materials functionality, further enabling the interplay between spatial resolution and noise levels. Having access to the full response data allows statistical explorations of the internal structure of the response in the frequency and information spaces using multivariate methods based on Principal Component Analysis (PCA). When dominant behaviour types are established, tools including two-dimensional (2D) correlation functions can: quickly identify underlying sources of observed behaviour; establish relationships between different responses; and enable further physics based data exploration in an objective and unbiased manner. Full information analysis in dynamic AFM As a basic paradigm of G-mode AFM we employ the concept of the multivariate analysis of the full cantilever response. The cantilever is driven by a suitably chosen excitation signal corresponding to conventional single frequency, dual frequency, band excitation or more complex excitation modes. However, unlike the heterodyne or parallel heterodyne processing in the classical AFM, in G-AFM the full response of the cantilever is captured and stored for each pixel and subsequently analysed and compressed for long-term storage. By ‘full response’ we imply that practically any available degrees of freedom, or information streams, can be recorded simultaneously on multiple channels. These can include vertical response, lateral response, and current. Stored data is then decorrelated, simplified and processed using appropriate multivariate methods and resulting data sets are visualized and analysed. Here we demonstrate G-mode AFM analogous to a standard intermittent (or tapping mode) AFM realized for simple sinusoidal driving. As a model material system we have chosen a spin-coated thin polymer film on mica consisting of 1:1 ratio of polystyrene and polycaprolactone. Additional experimental details can be found in the Methods section below. The corresponding surface topography and tapping mode amplitude and phase responses of the sample are shown in Fig. 1a–c . For G-mode, a separate data capturing software package was developed using Matlab and LabView, with all data post-processing performed in Matlab. Typically G-mode data were collected over 256 or 512 lines in the slow scan direction and continuous data collection within a line in either the trace or retrace direction. Typical raw data file sizes in G-mode for the conditions given above range from 4 to 8 GB, with an acquisition time per image of ~18 min. Here the microscope was operated in NAP (also known as interleave or lift mode, more details given in the Methods section) mode; the data was only captured during one of the four passes. Following the multivariate analysis and information-preserving compression, the data sets can be saved in the form of statistically relevant components typically ranging to the first thousand principal components, although depending on the system and imaging mode, further compression may be possible. Below, we discuss information processing of the full data set and discuss long-term storage later. 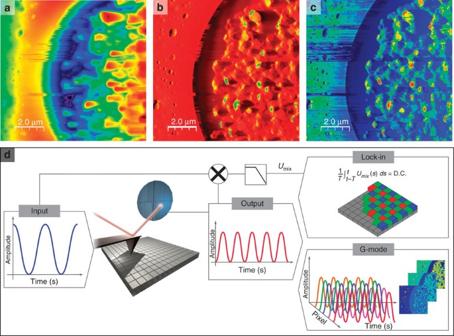Figure 1: G-mode compared to lock-in-based imaging. (a–c) Images collected over a single tapping mode scan with the feedback maintaining a set-point amplitude. (a) Single-frequency topography. (b) Single-frequency amplitude. (c) Single-frequency phase. (d) Lock-in and G-mode signal processing paradigms, lock-in integrates the mixed input/output signal over the time constant producing a single value (D.C. bias); G-mode captures the entire raw signal from the photodetector at each pixel, allowing different parameter map reconstruction. Figure 1: G-mode compared to lock-in-based imaging. ( a – c ) Images collected over a single tapping mode scan with the feedback maintaining a set-point amplitude. ( a ) Single-frequency topography. ( b ) Single-frequency amplitude. ( c ) Single-frequency phase. ( d ) Lock-in and G-mode signal processing paradigms, lock-in integrates the mixed input/output signal over the time constant producing a single value (D.C. bias); G-mode captures the entire raw signal from the photodetector at each pixel, allowing different parameter map reconstruction. Full size image When acquired and stored, the full response data can be initially processed in a manner similar to conventional AFM. For example, the magnitude of the ratio of the Fast Fourier Transform (FFT) of response to the FFT of the input signal at a given frequency (for example, driving frequency) produces cantilever response amplitude and phase similar to amplitude and phase images in conventional, LI amplifier-based AFM [17] . In addition, the full data set can be analysed and compressed using multivariate statistical methods, the underlying paradigm of G-mode AFM. Figure 1d illustrates the two archetypes, the top row of the schematic shows typical LI-based imaging, where both input and output signals to the cantilever produce only a single data point per pixel that has been averaged over the time constant of the amplifier. The bottom row depicts the G-mode approach, where the output waveform is stored in its entirety at each pixel allowing access to multiple cantilever modes and harmonics in their pure state, without mixing and scrambling or averaging and information loss. Note that the results of classical and G-mode analyses can be compared directly, as will be explored later. Analysis flow To systematically explore the full information contained in the tip–surface interaction, we apply multivariate statistical analysis to the cantilever response, to extract statistically significant contributions to the signal, organize them in the order of statistical significance, analyse intrinsic correlations and compress for long-term storage. The complete oscillation waveform is sliced into sequential time segments. In the simplest case, each segment is selected to match the spatial pixel time; however, the length can be varied allowing for multiresolution imaging (we refer to this as effective pixel). Thus obtained three-dimensional (3D) data set is decomposed in ordered statistically significant components through PCA [9] , [18] , [19] , [20] , [21] . In PCA, defined by equation (1) spectroscopic data set of N × M pixels populated by spectra containing P points is represented as a superposition of the eigenvectors w j , where a ik ≡ a k ( x, y ) are expansion coefficients at each pixel, A i ( t j )≡ A ( x , y , t j ) is the time dependence of cantilever response at selected spatial pixel, and t j are the discrete temporal points at which response is measured. The eigenvectors w k ( t ) and the corresponding eigenvalues λ k are calculated with a covariance matrix, C = AA T , where A is the matrix of all experimental data points A ij , that is, the rows of A correspond to individual grid points ( i =1,..., N × M ), and columns correspond to cantilever deflection over the time of that particular pixel, ( j =1,..., P ). Here note that the eigenvectors can be either plotted in time domains, or for convenience transferred into the Fourier domain. Since both PCA and FFT are linear operations, the FFT and PCA (before truncating of expansions) are commutative and hence eigenvectors can be explored in either time or frequency domains. The eigenvectors w k ( t ) are orthogonal and are chosen so eigenvalues are placed in descending order, λ 1 > λ 2 >..... Hence, the first eigenvector w 1 ( t ) contains the most information (where information is defined as variance) within the spectral-image data set; the second contains the most ‘informative’ (varying) response after the subtraction of the first one and so on. In this manner, the first p maps, a pk ( x, y ), contain the majority of information within the 3D data set, while the remaining P – p sets are dominated by noise. Shown in Fig. 2 is the result of PCA performed on a G-mode data set of the same area presented in Fig. 1 . In Fig. 2 , top row illustrates loading maps for the first four components. Additional components and their loadings can be found in the Supplementary Figs 1, 2 with a more in depth background discussion in the Supplementary Note 1 and first 50 eigenvectors with loadings in the Supplementary Movie 1 . The corresponding eigenvectors in the Fourier domain are shown in the bottom row, with inserts being the real space eigenvectors and selected real space zoomed in regions. It is clear that the first two PCA components are dominated by the information that is similar to the real and imaginary at the driving frequency shown in Fig. 1 . This conclusion is corroborated by the first two eigenvectors that show an approximately five order of magnitude stronger response at 73 kHz, that is, driving frequency. Here we note that for the simple harmonic oscillator model the first and second PCA components will be the sinusoidal signals shifted by 90° (since eigenvectors are orthogonal), hence corresponding to X and Y lock-in signals. Correspondingly, all other PCA components convey information beyond a single linear SHO response. For example, third and fourth eigenvectors in real space show characteristics of transient modulation behaviour attributed to the transients of cantilever oscillations induced by topography, that is, error in the feedback loop (note characteristic responses on the edges of topographic features). 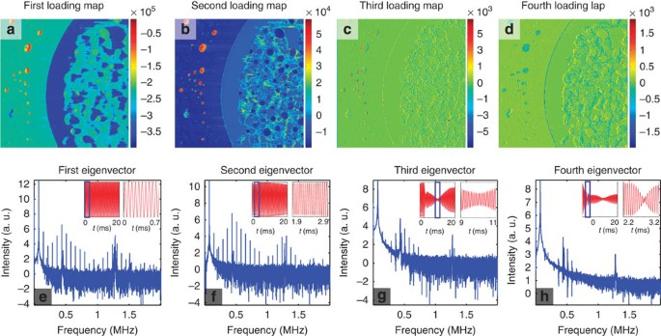Figure 2: Principal Component Analysis (PCA) loadings and eigenvectors as power density spectra and in real space. (a) Loading for the first eigenvector. (b) Loading for the second eigenvector. (c) Loading for the third eigenvector. (d) Loading for the fourth eigenvector. (e) Power spectral density of the First eigenvector with the inset showing the eigenvector in real space. (f) Power spectral density of the Second eigenvector with the inset showing the eigenvector in real space. (g) Power spectral density of the Third eigenvector with the inset showing the eigenvector in real space. (h) Power spectral density of the Fourth eigenvector with the inset showing the eigenvector in real space. Figure 2: Principal Component Analysis (PCA) loadings and eigenvectors as power density spectra and in real space. ( a ) Loading for the first eigenvector. ( b ) Loading for the second eigenvector. ( c ) Loading for the third eigenvector. ( d ) Loading for the fourth eigenvector. ( e ) Power spectral density of the First eigenvector with the inset showing the eigenvector in real space. ( f ) Power spectral density of the Second eigenvector with the inset showing the eigenvector in real space. ( g ) Power spectral density of the Third eigenvector with the inset showing the eigenvector in real space. ( h ) Power spectral density of the Fourth eigenvector with the inset showing the eigenvector in real space. Full size image Note the richness of the output signal elucidated by the Eigenvectors and corresponding loading maps, typically completely ignored in standard LI and PLLs. The driving frequency at 73 kHz, second cantilever mode at 435 kHz and third mode at 1.2 MHz are clearly present in all eigenvectors. These are visible as a result of thermal excitation and broad-band excitation resulting from tip–surface impact during tapping. In addition, harmonics of the driving frequency are present as well, along with mixed harmonic components. Digital LI calculations at those frequencies are trivial and are available from a single data set, providing readily available LI-like information at any frequency, examples are provided in Supplementary Figs 2, 3 as well as a Supplementary Movie 2 . An immediate advantage of collecting and storing an entire spectrum at each pixel location is the ability to inspect the sample response at each frequency response separately. As has been shown in Fig. 2 , the PCA eigenvectors indicate that even though the cantilever is driven at a single frequency, the response is rich with harmonics and higher modes. Fig. 3c,f illustrate what the response is at the second and third cantilever modes located at 435 kHz and 1.2 MHz, marked by red vertical lines. Fig. 3a,b,d,e are the corresponding simulated LI measurements at those response frequencies with the input frequency being the driving, at 73 kHz. While at 1.2 MHz there’s very little to no contrast, at 435 kHz, the signal is very strong and easily mapped. This information is invaluable for systems with behaviours occurring at different time scales. 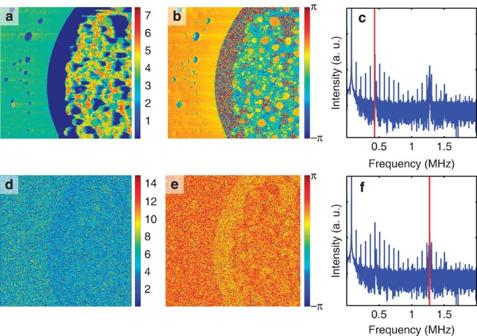Figure 3: Multifrequency lock-in illustration. (a) Amplitude image at 435 kHz. (b) Phase image at 435 kHz. (c) Location of the second mode at 435 kHz in the overall response, shown by a red line. (d) Amplitude image at 1.2 MHz. (e) Phase image at 1.2 MHz. (f) Location of the third mode at 1.2 MHz in the overall response, shown by a red line. Figure 3: Multifrequency lock-in illustration. ( a ) Amplitude image at 435 kHz. ( b ) Phase image at 435 kHz. ( c ) Location of the second mode at 435 kHz in the overall response, shown by a red line. ( d ) Amplitude image at 1.2 MHz. ( e ) Phase image at 1.2 MHz. ( f ) Location of the third mode at 1.2 MHz in the overall response, shown by a red line. Full size image We further proceed to analyse the spatial information present in the G-mode and frequency-dependent LI images. To quantify the contrast as the measure of spatially dependent signal, we calculate the radially averaged correlation function C ( r ) of images. By definition, C (0)=1. Here in the presence of discernible features the correlation function will have a long-range tail, whereas images populated by noise have rapidly decaying C ( r ), in the limit of random noise C ( r >0)=0. Fig. 4c illustrates the radial auto correlation function results for PCA produced images as a function of eigenvector, C ( r, n ). Note that the first three components contain discernible spatial features, whereas subsequent components contain either very short-range features (for example, topographic edges and so on) or are noise dominated. We pose that short-range features can be detected by exploring the correlations between the outliers of the image, but defer detailed analysis for future studies. Surprisingly, some of the senior components contain long-range correlations as well, as can be confirmed by visual inspection of the loadings maps. However, the full information is now contained in a relatively small number of modes. 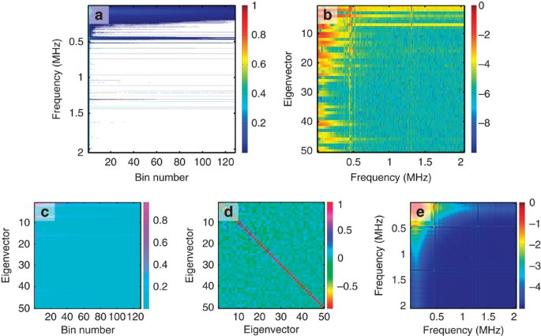Figure 4: Feature data mining, comparison of PCA to simulated lock-in results (LI). (a) Radially averaged correlation function results for images at each frequency, distributed over 128 bins. (b) 2D correlation function between the first 50 loadings and images at each measured frequency. (c) Radially averaged correlation function results for the first 50 loadings, distributed over 128 bins. (d) 2D self-correlation function results of the first 50 loadings. (e) 2D self-correlation function results of simulated LI images, absolute value of results with intensity on the log scale. Figure 4: Feature data mining, comparison of PCA to simulated lock-in results (LI). ( a ) Radially averaged correlation function results for images at each frequency, distributed over 128 bins. ( b ) 2D correlation function between the first 50 loadings and images at each measured frequency. ( c ) Radially averaged correlation function results for the first 50 loadings, distributed over 128 bins. ( d ) 2D self-correlation function results of the first 50 loadings. ( e ) 2D self-correlation function results of simulated LI images, absolute value of results with intensity on the log scale. Full size image Similar analysis for multifrequency LI is illustrated in Fig. 4a . In this case, the images with large scale features are clearly centred on the driving frequency and cantilever eigenmodes. However, the number of images containing this information is extremely large, and the information is spread over a large number of images and frequencies. We further proceed to explore the correlation between information contained between the G-mode and LI images, as depicted in Fig. 4b . To establish the similarity between mages, we use a cross-correlation coefficient defined in equation (2) as where A and B are input images and and are the 2D mean values of those images. The returned value r is the correlation coefficient between the two compared images and has a value of 1 to −1; where 1 means images correlate perfectly and −1 implies they are anticorrelated. Correlation coefficient of 0 suggests that images are independent. Results for the PCA loadings self-correlation are shown in Fig. 4d . These are the self-correlated loadings for each of the first 50 eigenvectors. Note that most of the off-diagonal elements are close to zero, suggesting that information in G-mode images is largely complementary and hence it allows for optimal representation of relevant features. For LI images, the correlation matrix is much more densely populated, Fig. 4e , suggesting that similar information is distributed over multiple images, inherently decreasing S/N ratio of individual images and hindering interpretation. Finally, the cross-correlation between G-mode and LI images are shown in Fig. 4b . Here the broad swaths of weak correlation peak in localized intensive peaks of excellent correlation and anticorrelation. In addition to identifying areas of interest and signal interplay in signal origins, these types of maps may hint at relative contributions of each of the frequencies to the response seen in PCA. Finally, G-mode AFM allows the analysis of the relevant information distribution in the combined frequency and information space. 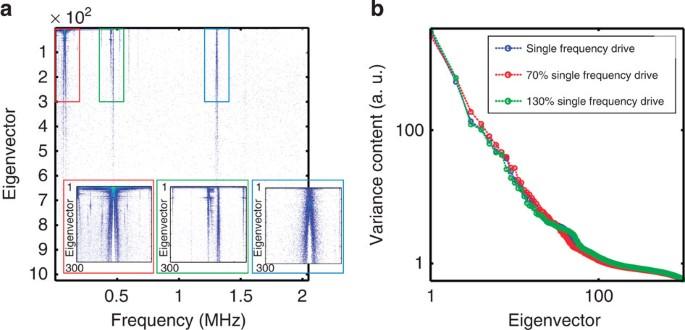Figure 5: Content of the captured data, a pathway to compression. (a) 2D representation of the first 1,000 eigenvectors as Power Density Spectra. (b) PCA Scree plot on a log–log scale. Figure 5a is a 2D representation of the FFT of the first one thousand eigenvectors (on the ordinate) plotted versus frequency (on the abscissa). The white background is set to the baseline noise average, so any pixels appearing are above the noise floor. The thickest vertical lines are three cantilever modes captured, with additional thinner lines being the harmonics of those modes. For the first 200 or so eigenvectors all the responses are highly pronounced and clear, those are the eigenvectors that contain variance related to the tip–surface interaction. Past 500, there are only faint traces of the response and after 700; information related to the cantilever vibrational modes is no longer available. Insets in the Fig. 5a highlight intricate doubling in the response of the vibrational modes, which we attribute to the statistics of single events and associated transients during imaging. A different metric of information relevance in PCA components is a Scree plot, (log–log plot of variance versus eigenvector number shown in Fig. 5b ), which shows the amount of variance in each eigenvector and is obtained during the PCA analysis. In Fig. 5b three lines represent different driving amplitudes for the G-mode method. The blue line labelled SF (single frequency) is the case of tapping amplitude of G-mode matching that of the microscope in standard AM–AFM operation (condition at which all presented data were collected). The red and green lines represent amplitude under drive and over drive, respectively. The figure illustrates that for these driving modes the information level past the hundredth eigenvector the slope of the line becomes constant before decreasing even further, signifying a significant drop in the information content. Figure 5: Content of the captured data, a pathway to compression. ( a ) 2D representation of the first 1,000 eigenvectors as Power Density Spectra. ( b ) PCA Scree plot on a log–log scale. Full size image In addition to providing insight into non-trivial information physics of data acquisition in dynamic AFM, this approach provides information on the limits of (loss less) information compression in G-mode. By definition, in PCA the number of eigenvectors has to be the same as the number of input spectra, as the method preserves the data and is reversible, which in the case of a 256 by 256 image should be the 256 [2] ; but since only the first 700 or so contain relevant information, only those 700 should be extracted and stored—allowing for low loss, and noise filtered, information compression by (in this case) almost two orders of magnitude. In other words, a 4 GB temporary file can be stored permanently at 40 MB containing essentially the same information (with some noise removed). At the same time, this analysis illustrates that statistically complete unbiased information requires these 700 components, not single-digit number of images. Information content in response components We note that complete loss-less information storage enabled by G-mode allows for detailed exploration of data in frequency and spatial domains. As an example of such analysis, we here introduce multiresolution imaging. Since each spatial pixel is now associated with a frequency response vector, the signal-to-noise (and/or frequency resolution) of the vector can be sacrificed to obtain higher spatial resolution. For example, if the original image is recorded at 256 × 256 pixels with 16,384 data points sampling the temporal response; this 3D data object can be converted to 256 × 2,048 pixels with 2,048 point sampling of the temporal response. In AFM this operation can be done in a single direction—the fast scanning direction, because there is no additional sampling in the direction of the slow scan axis. An example of multiresolution imaging is shown in Fig. 6 , panel (a) is a 256 × 256 resolution scan with a zoomed inset illustrating the edge resolution of a particular feature. Subsequent panels show the same feature, but at 256 × 1,024, 256 × 2,048 and 256 × 4,096 pixel resolutions. Perhaps the easiest place to see the compelling evidence to use this method is around the right boundary of the spherule feature. Initially, the boundary is defined by a single pixel with subsequent images showing a clearer shadow, some additional internal contrast and finally an internal halo preceding the border. Besides image clarity and higher quality pictures, this type of custom resolution allows examining features of interest in an image much more closely gaining additional insight that can be at far higher resolution. It is therefore possible to push the spatial information of an image to its noise limit, long after the measurement was taken. Additional information regarding force–distance curve information available in G-mode content is provided in the Supplementary Note 2 and Supplementary Figs 5, 6 . 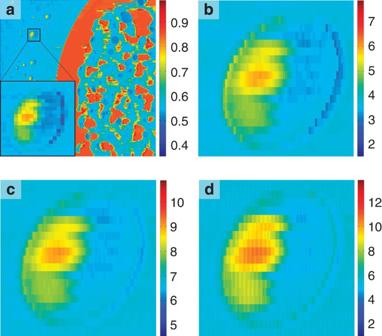Figure 6: Exploration of Multiresolution. (a) 256 × 256 image with a zoomed area of interest. (b) Area of interest from (a) at 256 × 1,024 resolution. (c) Area of interest from (a) at 256 × 2,048 pixels. (d) Area of interest from (a) at 256 × 4,096 pixels. Figure 6: Exploration of Multiresolution. ( a ) 256 × 256 image with a zoomed area of interest. ( b ) Area of interest from ( a ) at 256 × 1,024 resolution. ( c ) Area of interest from ( a ) at 256 × 2,048 pixels. ( d ) Area of interest from ( a ) at 256 × 4,096 pixels. Full size image Here we have introduced a novel concept for dynamic AFM data acquisition based on acquisition and multivariate analysis and compression of the entire response of the cantilever in time. The use of multivariate statistical methods such as PCA, allows one to guide a data sampling strategy and attain insight into how the data is structured in space, frequency and information domains. This method is much more advantageous compared with current LI-based techniques, since it provides a way to explore data without information loss or imposed bias, along with the statistical feedback to gain a complete understanding of a system, as well as effectively compress information to sought-after parameters of importance. Having access to the entire data set increases operator’s confidence in the observed phenomena since the resulting signal can be analysed from different perspectives providing an answer to a myriad of question relating to data veracity and experimental conditions. Armed with this new, in depth knowledge, dynamic AFM can begin to transition to models that are dictated by physics of tip surface interaction as imprinted in the recorded full cantilever response. From a purely experimental perspective, a visualization of material properties with the ability to and tune the interplay between the microscope resolution, acquisition time and resampling of the data, allows for an entirely new way to visualize and differentiate processes occurring at the tip–surface junction. Microcopy data acquisition These data and all G-mode data have been obtained on a Cypher AFM system (Asylum Research). Pt-Cr coated Multi-75EG AFM cantilevers (NanoAndMore) have been used for all imaging modes. In conjunction with the standard instrument hardware we have used a Digitizer and an Analog Waveform Generator cards, supported by PXI architecture, supplied by National Instruments. Imaging was done in the double pass mode (NAP, lift and equivalent), where the initial trace and retrace are performed using the microscope’s internal excitation scheme and a LI. Second set of trace and retrace is performed with the feedback disengaged, with the custom sine waveform supplied to the tip and the cantilever response collected at 4 MHz. All single frequency images were collected in amplitude modulated mode with an 800 mV set point at the first vibrational mode of the cantilever (~70 kHz) and collected using the IgorPro control software bundled with the instrument; additional image and postprocessed was done in WsXM [22] and Matlab. Amplitudes of the imaging and G-mode modes were matched. Samples The sample is a spin-coated polymer film on mica consisting of 1:1 ratio of polystyrene and polycaprolactone. How to cite this article: Belianinov, A. et al . Complete information acquisition in dynamic force microscopy. Nat. Commun , 6:6550 doi: 10.1038/ncomms7550 (2015).